Turbulence drives microscale patches of motile phytoplankton Patchiness plays a fundamental role in phytoplankton ecology by dictating the rate at which individual cells encounter each other and their predators. The distribution of motile phytoplankton species is often considerably more patchy than that of non-motile species at submetre length scales, yet the mechanism generating this patchiness has remained unknown. Here we show that strong patchiness at small scales occurs when motile phytoplankton are exposed to turbulent flow. We demonstrate experimentally that Heterosigma akashiwo forms striking patches within individual vortices and prove with a mathematical model that this patchiness results from the coupling between motility and shear. When implemented within a direct numerical simulation of turbulence, the model reveals that cell motility can prevail over turbulent dispersion to create strong fractal patchiness, where local phytoplankton concentrations are increased more than 10-fold. This ‘unmixing’ mechanism likely enhances ecological interactions in the plankton and offers mechanistic insights into how turbulence intensity impacts ecosystem productivity. Patchiness in the distribution of phytoplankton has long intrigued fishermen and scientists alike, because it generates hotspots of organisms at higher trophic levels [1] , [2] and modulates species diversity [3] , rates of fish recruitment [4] and population stability [5] . While phytoplankton patchiness at large spatial scales is driven by reproduction, growth is too slow to generate structure at scales 1 km vis-à-vis the homogenizing effect of turbulence [6] , [7] . Below this bottleneck scale, patchiness generated by locally enhanced growth is transferred to progressively smaller scales by turbulent stirring. Whereas traditional plankton sampling techniques that utilize nets and bottles average over scales of metres, new technologies, including high-resolution fluorometers [8] , [9] , underwater imaging [10] , [11] and syringe arrays [12] , offer vastly improved resolution of plankton distributions, and have revealed that the microscale (~1–10 cm) distribution of motile phytoplankton species (for example, dinoflagellates) is often considerably more patchy than the distribution of non-motile species (for example, diatoms) [10] , [11] , [12] . However, the mechanisms that underlie this observation have remained elusive. Here we show that phytoplankton motility, when occurring in a turbulent flow, generates intense patchiness, far exceeding that of randomly distributed, non-motile populations. H. akashiwo motility within a steady vortex flow Following the tradition of using a vortical flow as a first proxy for small-scale turbulence [13] , we exposed the motile, harmful algal bloom forming phytoplankter H. akashiwo to a steady vortex pair created via cavity flow ( Fig. 1a ; Methods). 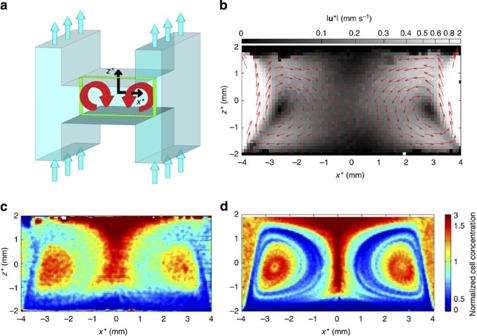Figure 1: Motility produces patchy phytoplankton distributions in a vortical flow. (a) An upward flow of a phytoplankton suspension (straight cyan arrows) past a central chamber was used to generate two counter-rotating vortices (curved red arrows).H. akashiwocells, illuminated by a laser sheet, were imaged along the central plane (green rectangle). (b) The flow fieldu* along the central plane of the chamber. Arrows denote fluid velocity and grey-scale intensity represents velocity magnitude. (c,d) Spatial distribution of phytoplankton cells in the central plane of the chamber fromcexperiments anddsimulations. Cell concentrations were normalized by the mean concentration (Supplementary Methods). AsH. akashiwodirects its motility opposite to gravity, cells that were able to escape the flow collected on the device’s upper boundary: we thus used a nonlinear colourmap to simultaneously visualize these surface aggregations and those within the vortex cores. In a control experiment, killed cells remained randomly distributed (Supplementary Fig. S2). Asterisks denote dimensional variables and gravity acts in the –zdirection. Video microscopy revealed that motile cells formed dense patches ( Fig 1c , Supplementary Movie 1 ). In addition to swimming into downwelling regions, as previously predicted [14] , [15] and observed in pipe flow [16] , they accumulated inside the vortices’ cores, showing that individual vortices can trigger striking patches of motile phytoplankton. In contrast, killed cells remained randomly distributed ( Supplementary Fig. S2 ), demonstrating that motility was an essential ingredient of patchiness. Figure 1: Motility produces patchy phytoplankton distributions in a vortical flow. ( a ) An upward flow of a phytoplankton suspension (straight cyan arrows) past a central chamber was used to generate two counter-rotating vortices (curved red arrows). H. akashiwo cells, illuminated by a laser sheet, were imaged along the central plane (green rectangle). ( b ) The flow field u * along the central plane of the chamber. Arrows denote fluid velocity and grey-scale intensity represents velocity magnitude. ( c , d ) Spatial distribution of phytoplankton cells in the central plane of the chamber from c experiments and d simulations. Cell concentrations were normalized by the mean concentration ( Supplementary Methods ). As H. akashiwo directs its motility opposite to gravity, cells that were able to escape the flow collected on the device’s upper boundary: we thus used a nonlinear colourmap to simultaneously visualize these surface aggregations and those within the vortex cores. In a control experiment, killed cells remained randomly distributed ( Supplementary Fig. S2 ). Asterisks denote dimensional variables and gravity acts in the – z direction. Full size image Motility is a pervasive trait of phytoplankton. For example, 90% of species forming harmful algal blooms can swim [17] . Motility allows cells to reside near the surface during daylight hours to enhance light acquisition while accessing deeper waters with more nutrients and lower predation risk at night [18] , [19] . To migrate through the water column, many species rely on a stabilizing torque that biases their swimming in the vertical direction [20] , [21] . This stabilizing torque competes with the viscous torque exerted on cells by fluid shear (specifically, the spatial gradients in fluid velocity that contribute to vorticity), which acts to overturn cells. The resulting directed motility is termed gyrotaxis, and the gyrotactic reorientation timescale, B —the characteristic time a perturbed cell takes to return to its vertical equilibrium orientation, k —provides a measure of how unstable the cell is to shear [20] , [21] , [22] . Gyrotactic motility within simulated flow fields The hypothesis that the observed patchiness ( Fig. 1c ) originated from the coupling of motility and the shear in the vortical flow is strongly supported by a mathematical model of gyrotactic motility [21] (Methods). When parameterized with the measured swimming properties of H. akashiwo , this model yields cell distributions in close agreement with experiments ( Fig. 1c ; Supplementary Fig. S4 ; Supplementary Movies 1 and 2 ). However, will patches of cells also occur in turbulent flow, where individual vortices are short-lived and the action of many vortices tends to disperse patchiness? To find out, we seeded a direct numerical simulation (DNS) of isotropic, homogeneous turbulence with up to 3.2 × 10 6 cells, whose motility was governed by the same model of gyrotaxis, and followed their trajectories until their spatial distribution reached a statistical steady state (Methods). We found that turbulence drives intense patchiness in the distribution of motile phytoplankton ( Fig. 2b ; Supplementary Movie 3 ), whereas non-motile cells follow the flow and remain randomly distributed ( Fig. 2a ). 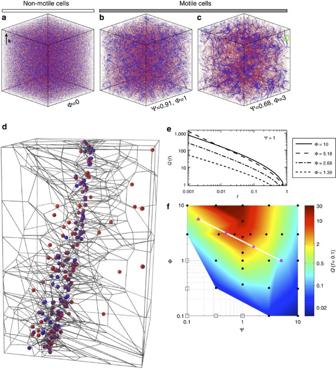Figure 2: Turbulence generates small-scale patchiness in the distribution of motile phytoplankton. (a–c) The positions of 300,000 cells swimming in a DNS of turbulent flow for three [Ψ, Φ] regimes. The 150,000 phytoplankton with the largest concentration (corresponding tof=0.5) are shown in blue, the remaining cells in red. Motile cells (b,c) exhibit strong patchiness, whereas non-motile cells (a) remain randomly distributed. (d) Three-dimensional Voronoi tessellation used to calculate the local cell concentration. Each cell is assigned the polyhedron that includes all points whose distance to that cell is smaller than its distance to any other cell. The inverse of the polyhedron’s volume is the cell concentration. The region shown corresponds to the green box inc. Cell colours are as ina–c, with cells in blue belonging to regions of higher cell concentration than cells in red. (e) The patch concentration enhancement factor,Q, measures the concentration of the most aggregated fractionfof cells relative to that of a non-motile (random) distribution, revealing that motility can drive the formation of patches with concentrations orders of magnitude larger than that of non-motile cells. (f) The cell concentration within patches,Q(here for the 10% most aggregated cells,f=0.1), increases with the non-dimensional swimming speed, Φ, and peaks at intermediate stability numbers, Ψ~1. The white line denotes the [Ψ, Φ] parameter space inhabited by a species withB=5 s andV=1,000 μm s−1swimming in a turbulent flow withε=10−6(pink square) and 10−9(pink triangle) m2s−3, and circular markers indicate 10-fold changes inε. Black circles and open squares are [Ψ, Φ] values at which simulations were performed. Open squares correspond to essentially random distributions (Q<0.01). Figure 2: Turbulence generates small-scale patchiness in the distribution of motile phytoplankton. ( a – c ) The positions of 300,000 cells swimming in a DNS of turbulent flow for three [Ψ, Φ] regimes. The 150,000 phytoplankton with the largest concentration (corresponding to f =0.5) are shown in blue, the remaining cells in red. Motile cells ( b , c ) exhibit strong patchiness, whereas non-motile cells ( a ) remain randomly distributed. ( d ) Three-dimensional Voronoi tessellation used to calculate the local cell concentration. Each cell is assigned the polyhedron that includes all points whose distance to that cell is smaller than its distance to any other cell. The inverse of the polyhedron’s volume is the cell concentration. The region shown corresponds to the green box in c . Cell colours are as in a – c , with cells in blue belonging to regions of higher cell concentration than cells in red. ( e ) The patch concentration enhancement factor, Q , measures the concentration of the most aggregated fraction f of cells relative to that of a non-motile (random) distribution, revealing that motility can drive the formation of patches with concentrations orders of magnitude larger than that of non-motile cells. ( f ) The cell concentration within patches, Q (here for the 10% most aggregated cells, f =0.1), increases with the non-dimensional swimming speed, Φ, and peaks at intermediate stability numbers, Ψ~1. The white line denotes the [Ψ, Φ] parameter space inhabited by a species with B =5 s and V =1,000 μm s −1 swimming in a turbulent flow with ε =10 −6 (pink square) and 10 −9 (pink triangle) m 2 s −3 , and circular markers indicate 10-fold changes in ε . Black circles and open squares are [Ψ, Φ] values at which simulations were performed. Open squares correspond to essentially random distributions ( Q <0.01). Full size image While marine turbulence is comprised of fluid motion at many scales, phytoplankton cells (~1–100 μm) only experience the shear from small scales where fluid viscosity dissipates energy. The characteristic size and shear rate of these dissipative scales are proportional to the Kolmogorov length scale, η K =(ν 3 /ε) 1/4 ~0.1–10 mm, and Kolmogorov shear rate, ω K =(ε/ν) 1/2 ~0.01–10 s −1 , respectively, where ν is the kinematic viscosity of seawater and ε the rate at which turbulent energy is dissipated [23] , [24] , [25] . Two dimensionless parameters then control the cells’ fate: the swimming number, Φ= V C / V K , measuring the swimming speed V C relative to characteristic small-scale fluid velocities V K = η K ω K =(νε) 1/4 (the Kolmogorov velocity), and the stability number, Ψ= Bω K , measuring how unstable upward swimming cells are to overturning by shear. We note that while most turbulent energy is dissipated by fluid motion with length scales larger than η K (ref. 23 ) the Kolmogorov scales remain the appropriate parameters for dimensionless analysis (Supplementary Fig. S8; Supplementary Methods). Through coupling with turbulence, motility can increase local cell concentrations by one or more orders of magnitude. To quantify local cell concentrations, we used a three-dimensional Voronoi tessellation [26] ( Fig. 2d ; Supplementary Methods ). The fraction f of cells having the largest local concentration were defined as patches and used to compute the patch concentration enhancement factor, Q= ( C — C P ) /C M , where C is the mean cell concentration within patches, C P is its counterpart for a random (that is, non-motile) distribution of cells (which also harbours fluctuations in cell concentration), and C M is the overall cell concentration. Thus, Q is a dimensionless measure of the increase in the local cell concentration due to motility. We found that motility can profoundly affect patch intensity. For example, the 10% most aggregated motile cells ( f =0.1) for Ψ=1 and Φ=2.68 were nearly 10 times ( Q =8) more concentrated than the 10% most aggregated non-motile cells ( Fig. 2e ). For the 1% most aggregated cells ( f =0.01), the enhancement is >50-fold ( Q =51). As patches are continuously born by motility and killed by turbulent dispersion, each cell transiently samples regions with high concentrations of conspecifics, on average spending a fraction of time f in regions where the local concentration is Q- fold larger than that of a random distribution. The patchiness intensity depends on both phytoplankton physiology and environmental conditions. Fast swimming cells (large Φ) with intermediate stability (Ψ~1) form the most concentrated patches ( Fig. 2f ). Owing to the incompressibility of the fluid, cells can form patches only if they swim across streamlines to converge within specific regions of the flow: they do so most effectively when their speed is large and their stabilizing torque strikes a balance between producing a swimming direction that is highly unstable and isotropic (Ψ>>1) and one that is very stable and uniformly upwards (Ψ<<1; Supplementary Fig. S9 ) [22] . Motility-driven unmixing generates strong patchiness for conditions that commonly occur in the ocean. The reorientation timescale, while known only for a handful of species [16] , [20] , [21] , [27] , [28] , [29] , generally spans the range B ~1–10 s, which, for typical turbulent dissipation rates (ε=10 −8 –10 −6 m 2 s −3 ), corresponds to Ψ~1. Phytoplankton swimming speeds [30] , [31] , V C ~100–1,000 μm s −1 , are often comparable to or larger than the Kolmogorov velocities, V K ~300–1,000 μm s −1 , associated with these dissipation rates, suggesting Φ can often be of order unity. Thus, we expect that phytoplankton routinely inhabit regions of the [Ψ, Φ] parameter space where patchiness is intense ( Fig. 2f ). Importantly, our results indicate that phytoplankton do not need to swim faster than the speed of large-scale turbulent fluctuations to defy the homogenizing effect of turbulent dispersion, as previously suggested [10] , they only need to swim at speeds comparable to Kolmogorov fluctuations. Which feature of turbulence is responsible for patchiness? In contrast to steady vortical flow, where multiple mechanisms produce patches [15] , in turbulent flow we found a consistent, strong correlation between cell location and downward flow velocity ( Fig. 3d ), suggesting that patchiness results from a dominant mechanism: cell focusing in local downwelling regions. This result generalizes previous observations of gyrotactic focusing in laminar downwelling flows [21] and is rationalized by a theoretical analysis of the compressibility of the cell velocity field v = u +Φ p (the superposition of flow velocity, u , and swimming velocity, Φ p , where p is the swimming direction and all velocities are non-dimensionalized by V K ). As v has non-vanishing divergence, (for Ψ << 1; where u z is the vertical component of u ; Methods), patches form ( ) where 2 u z >0, or equivalently in downwelling flow ( u z <0), because 2 u z and u z are negatively correlated ( Supplementary Fig. S7 ; Methods). Both of these predictions are in good agreement with simulations ( Fig. 3d ; Supplementary Fig. S6 ), suggesting our analytical results offer a rational, mechanistic framework to interpret how motile phytoplankton form patches in disordered flows. 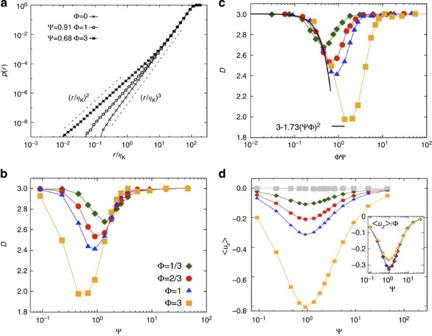Figure 3: Gyrotactic cells in a DNS of turbulence. Gyrotactic cells collect in downwelling regions, reducing the distance between neighbouring cells and triggering fractal patchiness. (a) Probabilityp(r) that two cells reside at a distance less thanrfrom each other. While at large scales (r>10ηK) the distribution of both non-motile (Φ=0) and motile (Φ>0) cells is volume-filling (p(r)~r3), at small scales (r<10ηK) motile cells exhibit fractal patchiness (p(r)~rDwithD<3). (b) The fractal dimensionDis smallest, corresponding to strongest patchiness, at intermediate stability numbers (Ψ~1) and large swimming speeds (large Φ). (c) The theoretical prediction of the fractal dimension,D=3–a(ΨΦ)2(Methods), accurately captures the simulation results for Ψ<1 (here,a=1.73 andr2=0.92). (d) The non-dimensional vertical fluid velocity averaged over the positions of all cells, <uz>,shows that populations with intermediate stability (Ψ~1) are more likely to reside in downwelling regions (<uz><0, coloured lines). This correlation increases with the swimming number, Φ. For comparison, there is no correlation with horizontal fluid velocities (grey symbols). (d, inset) Rescaling <uz> by Φ reveals that <uz> can reach ~30% of the swimming speed, reducing rates of upward migration. Figure 3: Gyrotactic cells in a DNS of turbulence. Gyrotactic cells collect in downwelling regions, reducing the distance between neighbouring cells and triggering fractal patchiness. ( a ) Probability p ( r ) that two cells reside at a distance less than r from each other. While at large scales ( r >10 η K ) the distribution of both non-motile (Φ=0) and motile (Φ>0) cells is volume-filling ( p ( r )~ r 3 ), at small scales ( r <10 η K ) motile cells exhibit fractal patchiness ( p ( r )~ r D with D <3). ( b ) The fractal dimension D is smallest, corresponding to strongest patchiness, at intermediate stability numbers (Ψ~1) and large swimming speeds (large Φ). ( c ) The theoretical prediction of the fractal dimension, D =3– a (ΨΦ) [2] (Methods), accurately captures the simulation results for Ψ<1 (here, a =1.73 and r 2 =0.92). ( d ) The non-dimensional vertical fluid velocity averaged over the positions of all cells, < u z >, shows that populations with intermediate stability (Ψ~1) are more likely to reside in downwelling regions (< u z > <0, coloured lines). This correlation increases with the swimming number, Φ. For comparison, there is no correlation with horizontal fluid velocities (grey symbols). ( d , inset) Rescaling < u z > by Φ reveals that < u z > can reach ~30% of the swimming speed, reducing rates of upward migration. Full size image Motility substantially decreases the distance between neighbouring phytoplankton cells, altering the topology of their distribution. We found that the probability p ( r ) that a pair of cells reside less than a distance r from each other is enhanced for r <10 η K and this enhancement is >100-fold for r <0.2 η K (for Ψ=0.68, Φ=3; Fig. 3a ). For ε =10 −6 m 2 s −3 ( η K ~1 mm), this translates to a >100-fold increase in the probability that a conspecific resides within ~200 μm of a given cell. Whereas non-motile cells are randomly distributed in three-dimensional space, with p ( r ) ~r 3 , for motile cells we found that p ( r ) ~r D with D <3 ( Fig. 3a ), signifying that the cell distribution is not volume-filling, but instead occupies a lower-dimensional fractal set [32] . Fractal clustering of particles in fluids is well known, for example in particles floating on fluid surfaces [33] and water droplets in clouds [34] , and arises as a consequence of an effective compressibility, which here stems from the ability of cells to swim across streamlines. Our analysis of the divergence of v correctly predicts the patchiness topology: weakly compressible flows are expected to produce particle distributions residing on a fractal set of codimension D =3 − a (ΨΦ) [2] , where a is a constant and Ψ<<1 (Methods and Falkovich et al. [34] ). This relation successfully captured the behaviour of the fractal dimension D computed from simulations for Ψ<1 ( Fig. 3c ), confirming that the interaction of motility and turbulent flow results in an effective compressibility, which generates patchiness. Patchiness generated by motility-driven unmixing may have a multitude of consequences for phytoplankton. On the one hand, patchiness may be advantageous during times of sexual reproduction, as it reduces distances between conspecific cells and could increase the local concentration of phytoplankton-exuded toxins that stifle competitors [35] . On the other hand, patchiness could be detrimental because it sharpens competition for nutrients [36] and enhances grazing by zooplankton [37] , [38] , whose finely tuned foraging strategies allow them to retain their position within centimeter-scale prey patches [2] . The interaction of motility and turbulence could thus be an important determinant of the relative success of different phytoplankton species and provide a mechanistic basis to help decipher the powerful role turbulence is known to exert on plankton community composition [39] . Unlike passive mechanisms that generate patchiness, such as turbulent stirring, motility-driven unmixing stems from active cell behaviour, opening the intriguing possibility that phytoplankton could regulate their small-scale spatial distribution by adaptively adjusting their position in [Ψ, Φ] space ( Fig. 2f ). Cells could regulate Φ by modulating swimming speed and Ψ by altering flagellar stroke [20] , overall shape [40] or chloroplast position [41] . Individuals could then actively increase encounter rates with conspecifics, without need for chemical communication, by swimming faster and tuning stability such that Ψ~1, or minimize predation risk by slowing down and avoiding the intermediate stability regime. Regardless of whether this mechanism is adaptive or static, these results suggest that small-scale patchiness is a corollary of vertical phytoplankton migration, and that motility-driven patch formation may thus be as common as the species that migrate through the water column. Future field and laboratory experiments may reveal the tradeoffs of directed motility in a turbulent ocean and how it shapes the fate of those at the bottom of the marine food web. Phytoplankton culturing and preparation H. akashiwo was grown by inoculating 2 ml of exponential phase culture into 25 ml of sterile f/2 medium, then incubating at 25 °C under continuous fluorescent illumination (70 μE m −2 s −1 ) for 21 days. The culture used in experiments was prepared by diluting 75 ml of the 21-day old culture with 500 ml of f/2 media to achieve a final cell concentration of ~2.5 × 10 4 cells ml −1 . This concentration strikes a balance between maximizing the number of cells within the central plane ( Fig. 1a , green box) and avoiding the bioconvective instabilities that arise when cell concentration exceeds a critical threshold [21] . In control experiments ( Supplementary Fig. S2 ), cells were killed using ethanol (10% v/v) before their introduction into the device. Experimental vortex apparatus Two counter-rotating vortices were generated within a custom-made transparent acrylic device ( Fig. 1a and Supplementary Fig. S1 ). A 0.3 ml s −1 flow of a H. akashiwo culture was driven through each of the two vertical channels of the device using a syringe pump (Harvard Apparatus, PHD 2000) loaded with two syringes (Monoject, 140 ml). A random distribution of cells was initialized within the central cavity of the device ( Fig. 1a , green box) by clamping one of the two flexible tubes (Cole Parmer C-Flex, ID 3 mm) that convey flow to the device, which induced a unidirectional flow through the central cavity. Once the tube was unclamped, vortical flow was restored and the experiment began. A laser sheet, generated using a continuous wave 8 mW Helium-Neon laser (Uniphase, model 1105 P) and a plano-concave cylindrical lens (Thorlabs, 20 mm focal length), illuminated cells along a 1.6-mm thick central plane (−0.8 mm< y * < 0.8 mm, where the asterisk denotes a dimensional variable) where the flow was nearly two-dimensional due to symmetry. All images were captured at 20 Hz with a CCD (charge-coupled device) camera (PCO 1600, Cooke) attached to a dissecting microscope (SMZ1000, Nikon). Simulations of gyrotaxis within the experimental flow field To model the flow within the experimental device, we solved the three-dimensional Navier-Stokes equations with the finite element software COMSOL Multiphysics (Burlington, MA), using the experimental device’s exact geometry and imposed flow rates. Gyrotactic motility was modelled by integrating the equation for the evolution of the swimming direction of a bottom-heavy spherical cell [21] where p is the unit vector along the swimming direction, ω *= * × u * is the fluid vorticity, t * is time, k =[0,0,1] is a unit vector in the vertical upwards (+ z *) direction, and B is the gyrotactic reorientation timescale, the characteristic time a perturbed cell takes to return to vertical if ω *=0. The first term on the right hand side describes the tendency of a cell to remain aligned along the vertical direction due to bottom-heaviness, while the second term captures the tendency of vorticity to overturn a cell by imposing a viscous torque on it. We neglect the effect of cells on the flow. The cell position, X *=( x *, y *, z *), was computed by integrating the velocity resulting from the superposition of the swimming velocity, V C p , and the flow velocity, u *: Cell positions and swimming directions were initialized at random locations within the device and randomly on a unit sphere, respectively. Reflective boundary conditions were applied at all solid boundaries. The swimming speed, V C , of each cell was drawn from a probability distribution obtained from H. akashiwo cells swimming within the central plane of the experimental device in the absence of flow. Cell trajectories were obtained from movies recorded at 20 Hz using automated software (PredictiveTracker; Ouellette et al. [42] ). To estimate the three-dimensional swimming velocity from its measured ( x *, z *) projection, we assumed isotropy in x* and y * to obtain V C =(2 v x * 2 + v z * 2 ) 1/2 where v x * and v z * are the instantaneous cell swimming speeds in the x * and z * direction, respectively. The resulting probability density for the cell swimming speed has a mean of 75 μm s −1 ( Supplementary Fig. S3 ). All 70,000 cells used in the simulation had a gyrotactic reorientation parameter of B =2 s, based on a previous estimate for H. akashiwo [27] . Simulations of gyrotaxis within isotropic turbulence We solved the three-dimensional Navier-Stokes equations in a fully periodic cubic domain of size L B =2 π with M mesh points using a pseudo-spectral method with a vector potential representation to ensure fluid incompressibility [43] . To eliminate aliasing errors, we used the 2/3 dealiasing technique, which sets the largest 1/3 of all wave numbers to zero after each computation of the nonlinear terms in the Navier-Stokes equation [44] , such that the largest resolved wavenumber is k max =(1/3) M 1/3 . Statistically stationary turbulence was sustained by applying homogeneous, isotropic, time-uncorrelated Gaussian forcing over a narrow shell of small wavenumbers [45] , which produces integral-scale fluid fluctuations (that is, the size L of the largest eddy) on the order of the domain size. Once the velocity field had reached a statistical steady state, gyrotactic cells were initialized with random position in the domain and with orientations randomly distributed over the unit sphere. We seeded the simulation box with 300,000–3,200,000 cells depending on the Taylor Reynolds number Re λ ( Supplementary Table S1 ; Supplementary Methods ). Cell trajectories were integrated using the non-dimensional form of equations 1 and 2, where time was non-dimensionalized by 1/ ω K , lengths by the Kolmogorov length scale η K and velocities by the Kolmogorov velocity V K =ω K η K . Dimensionless parameters are Φ= V C / V K and Ψ= Bω K ( ω K is the Kolmogorov vorticity scale). At each time step of the simulation, the local fluid flow properties ( ω and u ) at the particle locations were calculated using a tri-linear interpolation from the computational mesh points. Previous studies have demonstrated that the trajectories of passive tracer particles integrated via this numerical scheme accurately capture both the velocity [46] and the acceleration [47] statistics of the underlying DNS-derived flow. Moreover, previous studies on clustering of inertial particles [48] have demonstrated the efficacy of this method to resolve sub-Kolmogorov scale fractal aggregations, which we also observed for gyrotactic swimmers. All analyses were performed after cells had reached a statistically steady distribution, which requires ~30–50 Kolmogorov time scales (1/ ω K ), corresponding in our simulations to 1–2 integral time scales (the characteristic timescale of the largest eddies in the flow). Theoretical prediction of accumulation in downwelling regions In general, the cell velocity field, v=u +Φ p , and its divergence, · v , depend on the history of the trajectory of individual cells and can only be calculated statistically. However, in the limit of a large stabilizing torque (Ψ<<1) the cell orientation quickly reaches equilibrium with the local fluid vorticity, such that v can be directly calculated using the instantaneous flow field. Assuming Ψ<<1, the solution to equation 3 is to leading order in Ψ. This predicts that cells swim upwards with a deviation proportional to Ψ from the vertical. Imposing the incompressibility of the flow ( · u =0) and applying the definition of vorticity, substitution of equation 5 into equation 4 yields where u z is the vertical component of fluid velocity, normalized by the Kolmogorov velocity, V K . Equation 6 predicts that the cell velocity is compressible and that aggregations form in regions where 2 u z >0. This prediction was confirmed in the DNS simulations by calculating ‹ 2 u z ›, defined as the mean of 2 u z at the position of the cells ( Supplementary Fig. S6 ). We found that ‹ 2 u z › reaches a maximum for Ψ~1 and increases monotonically with Φ, which mirrors the dependence of the aggregation intensity on Ψ and Φ ( Figs 2f and 3b ; Supplementary Fig. S6 ), indicating that cells form patches in regions where ‹ 2 u z › is large. The prediction that cells collect where 2 u z >0 generalizes prior observations that gyrotactic cells tend to collect in downwelling flows [21] , because regions of the flow where 2 u z >0 tend be highly correlated with regions of downwelling ( u z <0). This correlation can be demonstrated either by analysing the results from the DNS ( Supplementary Fig. S7 ) or via theoretical analysis. The latter is briefly outlined here. By recasting the Navier-Stokes equations as an energy balance one can write [25] where all variables are dimensional (asterisks omitted for brevity), ε is the average energy dissipation rate and the last equality assumes isotropic flow. We can then rewrite the averaged quantity in the last term as: where ‹ 2 u z |u z =u› is a conditional average and P ( u ) is the probability density distribution of a single component of the flow velocity field at a fixed point, which for turbulent flows is well approximated by the following Gaussian distribution [25] : Using a closure theory that assumes homogeneous, isotropic turbulent flow [49] , the conditional average in equation 8 can be approximated, to leading order, as Equation 10 is obtained by using a linear approximation for the conditional average and substituting equation 9 into equation 8 and the result into equation 7 (ref. 49 ). The relation in equation 10, which shows good agreement with our simulations ( Supplementary Fig. S7 ) predicts that, on average, regions with positive 2 u z are correlated with downwelling flow ( u z <0), and vice versa. These two predictions, that is, that cells collect where 2 u z >0 and that 2 u z ~− u z , taken together, indicate that an effective compressibility in the cell velocity field (produced by the cells’ motility) results in the formation of patches within downwelling regions, rationalizing the results from the turbulence simulations. Theoretical prediction of D In the previous section we showed that the cell's velocity field v has non-vanishing divergence in the limit of a strong stabilizing torque (Ψ<<1). In this limit, cells behave as passive tracers transported by a weakly compressible flow, v=u + δ w with · w =− 2 u z and δ =ΨΦ (equation 6). It has been previously shown that tracers in weakly compressible flows ( δ <<1) tend to form transient clusters of fractal codimension (3− D ) ∝ δ 2 (refs 34 , 50 , 51 , 52 ). Thus for gyrotactic swimmers with Ψ<<1, the fractal dimension is predicted as where a is a constant that depends on the flow. This result is in good agreement with our simulations for Ψ<1 ( Fig. 3c ). How to cite this article: Durham W. M. et al. Turbulence drives microscale patches of motile phytoplankton. Nat. Commun. 4:2148 doi: 10.1038/ncomms3148 (2013)